A bistable genetic switch based on designable DNA-binding domains Bistable switches are fundamental regulatory elements of complex systems, ranging from electronics to living cells. Designed genetic toggle switches have been constructed from pairs of natural transcriptional repressors wired to inhibit one another. The complexity of the engineered regulatory circuits can be increased using orthogonal transcriptional regulators based on designed DNA-binding domains. However, a mutual repressor-based toggle switch comprising DNA-binding domains of transcription-activator-like effectors (TALEs) did not support bistability in mammalian cells. Here, the challenge of engineering a bistable switch based on monomeric DNA-binding domains is solved via the introduction of a positive feedback loop composed of activators based on the same TALE domains as their opposing repressors and competition for the same DNA operator site. This design introduces nonlinearity and results in epigenetic bistability. This principle could be used to employ other monomeric DNA-binding domains such as CRISPR for applications ranging from reprogramming cells to building digital biological memory. Multistability is a widespread natural phenomenon in diverse biological processes, ranging from cell differentiation to the response to environmental signals. The basic feature of bistable systems is that once an input signal reaches a defined threshold value, the system switches into the corresponding stable state and remains in that state even after this signal is removed. Switching back to the initial state requires the pulse of a second input signal. Flip-flop (or SR latch) bistable switches represent the basic elements of finite-state machines composed of sequential logic circuits and the building blocks of memory storage elements in electronic circuits. In biological systems, genetic toggle switches play important roles in cell cycle progression, embryonal development, cancer, apoptosis and many other processes [1] , [2] , [3] , [4] , [5] , [6] . A basic engineered genetic toggle switch consists of two operons encoding a pair of repressors that mutually inhibit one another’s transcription [7] . This type of design for a genetic toggle switch has been implemented in bacteria [8] as well as in mammalian cells [9] . Although several natural prokaryotic transcription factors have been used to assemble genetic circuits [8] , [9] , [10] , [11] , the number of orthogonal transcription factors for the toolbox should be expanded to construct complex designed genetic circuits. Furthermore, the diverse biochemical properties of natural repressors may require adjustments to their strength and orthogonality to make them suitable for designed circuits [12] . A systematic approach for constructing bistability based on designed regulatory elements is needed. Modular DNA-binding domains are powerful tools for engineering synthetic cellular regulatory networks because these domains allow the plug-in combinations of DNA-binding and transcriptional effector domains. The DNA-binding domains of zinc finger proteins, transcription-activator-like effectors (TALEs), or CRISPR/Cas nuclease can be genetically fused to transcriptional effector domains to function as designed site-specific transcriptional activators or repressors targeted against almost any DNA sequence [13] , [14] , [15] , [16] , [17] , [18] , [19] , [20] . The ability to design these synthetic transcription factors to target a large sequential diversity of DNA operators should support the construction of complex designed genetic circuits. Recently, a complete set of static two-input logic gates based on designed TALE repressors was demonstrated in mammalian cells [21] . It would be desirable to use designable, orthogonal building elements such as TALEs as building blocks in the construction of dynamic, time-dependent logic systems, such as bistable switches. However, one potential problem of designed DNA-binding domains, such as TALEs, zinc finger proteins or CRISPR/Cas nucleases, lies in the monomeric nature of their binding to DNA. Systems theory concludes that a nonlinear response is essential for the functionality of multistable switches [9] , [22] . In cases of designed bistable switches implemented up to now, this has been achieved via the application of natural transcription factors that bind as oligomers to the operator DNA. The oligomerization of natural transcription factors evolved separately for each protein, which prevents a systematic modular engineering of orthogonal switches employing the same principles used to construct static logic gates. Therefore, the challenge is to introduce a nonlinear response into a system composed of orthogonal regulators with a linear response introducing a general principle that could be applied across different chassis and for different designable DNA-binding domains. Here we present a strategy for constructing bistable toggle switches based on designed monomeric DNA-binding domains. We demonstrated that the conventional design of a genetic toggle switch constructed from orthogonal TALE-based repressors did not result in a bistable system. A mathematical model of this design, based on experimentally determined parameters, showed that this was due to the non-cooperativity of TALE domain binding to DNA. Nonlinearity was introduced into the design via the introduction of activators and repressors based on the same DNA-binding domain. Those regulatory elements were wired to introduce competition for the DNA-binding site between an activator and a repressor, and to introduce positive feedback loops. The modelling and experimental validation of this genetic circuit design in human cell lines demonstrate the epigenetic stability of each of the two states of the switch and multiple toggling between the two states via induction by chemical signals, and provides the basis for the scalability for generating multiple switches and more complex logic circuits. Toggle switch based on two TALE repressors is not bistable Our initial goal was to prepare a mutual repressor switch comprising a pair of designed orthogonal TALE domain-based repressors and test its bistability in mammalian cells. The designed repressors were constructed via fusion of the selected TALE DNA-binding domains with the KRAB chromatin-silencing domain [23] . The position of the KRAB repression domains relative to the DNA-binding domain was investigated to determine the optimal arrangement of the effector domain regarding the DNA-binding domain ( Supplementary Fig. 1a,b ). Multiple copies of the binding site upstream from the promoter were used [21] to decrease the off-target effects and enhance the efficiency of repression. This resulted in up to 98% transcriptional repression, while the two selected TALE domains were mutually orthogonal and exhibited virtually no cross-talk ( Supplementary Fig. 1a,b ). To implement the toggle switch, the TALE repressor coding region fused to the carboxy-terminal KRAB domain was positioned under the control of the opposing DNA operator ( Fig. 1a ). Two fluorescent reporters, blue fluorescent protein and monomeric citrine protein, were genetically fused to each of the repressor operons via the t2A peptide linker [24] to help monitor the expression of each repressor in individual cells. For the external time-dependent selection of each of the two states, we introduced an input layer to regulate the transcription of selected TALE repressors under the control of chemical inducers (that is, pristinamycin and erythromycin) [25] , [26] ( Fig. 1b and Supplementary Fig. 1c,e ). The pristinamycin- and erythromycin-inducible systems coupled to the TALE repressors exhibited low leakage and an approximately fivefold difference in reporter expression between the stimulated and unstimulated states ( Supplementary Fig. 1d,f ). Experimental results regarding the TALE repressors and the induction layer provided parameters for the mathematical model ( Supplementary Notes 1 and 2 ). The complete setup of the TALE-based mutual repressor switch consisted of the induction layer regulating two mutual repressors, TALA:KRAB and TALB:KRAB ( Fig. 1b ). However, stimulation of mammalian cells transiently transfected with plasmids for this switch setup with either of the two chemical inducers degenerated into a simultaneous expression of both reporters, suggesting that this system cannot retain the stable state (data not shown). As an additional test, we examined cells with transiently introduced genetic switch circuit plasmids in the absence of external chemical induction. In a bistable system, each individual cell would be expected to adopt one of the two stable states based on the stochastic variations of each repressor level or based on the previous state of each cell. However, fluorescence microscopy analysis demonstrated that the majority of cells expressed both reporters within each cell simultaneously ( Fig. 1b ). We could not distinguish between the simultaneous transcription of both reporters and dynamic switching between both states in individual cells. Nevertheless, both explanations lead to the conclusion that this design of a mutual TALE-repressor-based genetic circuit is not bistable. 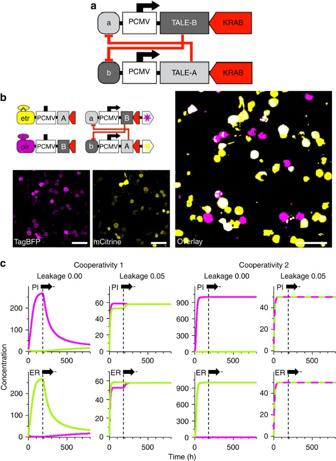Figure 1: The mutual repressor switch topology based on TALE repressors does not exhibit bistability. (a) The mutual repressor switch topology, consisting of two TALE repressor genes placed downstream of the constitutive CMV promoter with an operator for the opposing TALE repressor upstream of the promoter, and (b) TALE-based toggle with additional constructs for the external control and two different fluorescent protein reporters. The overlay of the microscopy images of the TALE-based mutual repressor switch indicates the simultaneous expression of both fluorescent reporter proteins in individual cells in the absence of external regulation. The images are representative of at least three independent experiments. Cells expressing TagBFP or mCitrine reporter genes are displayed in magenta or yellow, respectively. Cells expressing both reports at the same time (53%) are coloured white on the overlay image. Scale bar, 50 μm. The mCitrine and TagBFP reporters were linked to the repressor operons via the t2A peptide linker. For external switch control, the pristinamycin- and erythromycin-inducible transcriptional repressors (PIP:KRAB and E:KRAB, respectively) were added along with the pristinamycin- and erythromycin-inducible transcriptional control of the same pair of TALE repressors. (c) The deterministic modelling of the mutual repressors’ topology indicates that this setup can achieve state stability only with cooperative elements. The models of the non-cooperative systems did not result in state stability, even with high transcriptional repression as described inSupplementary Note 1. PI and ER stand for pristinamycin and erythromycin induction, respectively. Magenta and green lines indicate the calculated TagBFP and mCitrine reporter gene expression levels, respectively. Figure 1: The mutual repressor switch topology based on TALE repressors does not exhibit bistability. ( a ) The mutual repressor switch topology, consisting of two TALE repressor genes placed downstream of the constitutive CMV promoter with an operator for the opposing TALE repressor upstream of the promoter, and ( b ) TALE-based toggle with additional constructs for the external control and two different fluorescent protein reporters. The overlay of the microscopy images of the TALE-based mutual repressor switch indicates the simultaneous expression of both fluorescent reporter proteins in individual cells in the absence of external regulation. The images are representative of at least three independent experiments. Cells expressing TagBFP or mCitrine reporter genes are displayed in magenta or yellow, respectively. Cells expressing both reports at the same time (53%) are coloured white on the overlay image. Scale bar, 50 μm. The mCitrine and TagBFP reporters were linked to the repressor operons via the t2A peptide linker. For external switch control, the pristinamycin- and erythromycin-inducible transcriptional repressors (PIP:KRAB and E:KRAB, respectively) were added along with the pristinamycin- and erythromycin-inducible transcriptional control of the same pair of TALE repressors. ( c ) The deterministic modelling of the mutual repressors’ topology indicates that this setup can achieve state stability only with cooperative elements. The models of the non-cooperative systems did not result in state stability, even with high transcriptional repression as described in Supplementary Note 1 . PI and ER stand for pristinamycin and erythromycin induction, respectively. Magenta and green lines indicate the calculated TagBFP and mCitrine reporter gene expression levels, respectively. Full size image Although most natural transcription factors bind to DNA as oligomers (that is, dimers or tetramers), the crystal structure of the TALE DNA-binding domain clearly shows that it binds to the target DNA as a monomer [27] , [28] ; thus, the cooperativity of binding should be low. The same argument is also valid for other designable DNA-binding domains such as zinc finger- and CRISPR/Cas-based repressors. Deterministic models of the TALE-based mutual repressor switch demonstrated that this system could not retain the stable state and drifted to the mixed state ( Fig. 1c and Supplementary Note 1 ). Even in the case of the cooperativity coefficient of 2, this type of switch is sensitive to as little as 5% incomplete repression. Introduction of nonlinearity using monomeric binding domains The theoretical solution of introducing nonlinearity into a system composed of monomeric DNA-binding elements proposed the introduction of a pair of hypothetical transcription factors, each of which should be able to activate its own expression and simultaneously repress the transcription of the opposing transcription factor [29] , [30] . Such types of transcription factors would be very difficult to design. However, the modularity of the designed transcription factors allows the construction of a transcriptional activator or repressor, each targeting the same DNA-binding sequence, by coupling the DNA-binding domain to either the VP16 transactivation domain ( Supplementary Fig. 2a,b ) or the KRAB repression domain, respectively. We reasoned that such a pair of transcriptional regulators based on TALEs could be used to introduce nonlinearity into the designed switch circuit using two strategies: (a) the introduction of positive feedback loops and (b) competition between an activator and a repressor for the same DNA operator binding site. Simulations of a cellular circuit employing TALE activators and repressors wired to bind to separate DNA sites upstream from the promoter, thus without competition effects ( Fig. 2a ), did not result in bistability ( Fig. 2b and Supplementary Note 2 ). As the designed TALE-based repressor and activator can be based on the same DNA-binding domain, they could compete for binding to the target DNA site ( Fig. 3a ). The relative occupancy of the binding site and the resulting gene transcription should therefore depend on the ratio of the repressor and the activator, as they comprise the same DNA-binding domain ( Fig. 3b ). We performed simulations of the designed circuit using competition between TALE-based repressors and TALE DNA-binding domains without an effector domain ( Fig. 2c ), which demonstrated the functional bistability of this switch circuit topology ( Fig. 2d and Supplementary Note 2 ). This shows that the competition between the activator and the repressor for the same DNA site is an essential feature for introducing nonlinearity into a genetic circuit based on non-cooperative regulators. 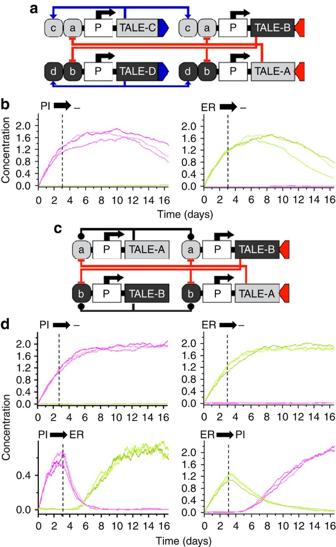Figure 2: Stochastic models demonstrate that competition for the binding sites between an activator and a repressor is an essential feature required for the bistability of the switch based on the monomeric binding of transcription factors. (a) Introduction of a positive feedback loop into the TALE-based mutual repressor switch by the addition of two TALE activator genes. Each of the TALE activators controls expression of its own gene and the corresponding repressor gene, while the latter also inhibits expression of the opposing TALE activator. Each TALE activator or repressor in this setup has a unique DNA-binding domain, eliminating the competition between activators and repressors. (b) Simulations of this genetic circuit demonstrate that the addition of a positive feedback loop is not sufficient for state stability. Details of the model are available inSupplementary Note 2. (c) Introduction of binding competition into the TALE-based toggle switch by the introduction of two TALE domains without regulatory domains. Each of the introduced TALE DNA-binding domains can bind to its own operon and to the operon of the opposing TALE repressor, introducing competition but not exerting direct operon activation or repression. (d) Simulations of this topology reveal that competition for binding sites is sufficient for the switch to assume a stable state in the presence of an inducer molecule. Details on the model are available inSupplementary Note 2. Figure 2: Stochastic models demonstrate that competition for the binding sites between an activator and a repressor is an essential feature required for the bistability of the switch based on the monomeric binding of transcription factors. ( a ) Introduction of a positive feedback loop into the TALE-based mutual repressor switch by the addition of two TALE activator genes. Each of the TALE activators controls expression of its own gene and the corresponding repressor gene, while the latter also inhibits expression of the opposing TALE activator. Each TALE activator or repressor in this setup has a unique DNA-binding domain, eliminating the competition between activators and repressors. ( b ) Simulations of this genetic circuit demonstrate that the addition of a positive feedback loop is not sufficient for state stability. Details of the model are available in Supplementary Note 2 . ( c ) Introduction of binding competition into the TALE-based toggle switch by the introduction of two TALE domains without regulatory domains. Each of the introduced TALE DNA-binding domains can bind to its own operon and to the operon of the opposing TALE repressor, introducing competition but not exerting direct operon activation or repression. ( d ) Simulations of this topology reveal that competition for binding sites is sufficient for the switch to assume a stable state in the presence of an inducer molecule. Details on the model are available in Supplementary Note 2 . 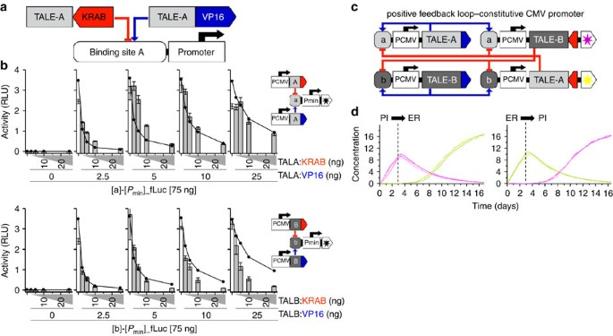Figure 3: Introduction of nonlinearity into a genetic circuit based on monomeric DNA-binding elements employing competition and positive feedback loops. (a) A TALE repressor and a TALE activator based on the same DNA-binding domain competing for binding to the same DNA target site. (b) The competition of the TALE-based activator and repressor for the same binding site was experimentally tested using the luciferase reporter. Various ratios of plasmids constitutively expressing a TALE activator and a TALE repressor based on the same DNA-binding domain were co-transfected into HEK293T cells, along with 75 ng of the corresponding reporter plasmid, which resulted in different levels of the expression of the reporter. The values represent the mean and s.d. of three replicates and are representative of at least three independent experiments. Fit of the model based on parameters extracted from the experimental data of all experiments overlays the experimental data. (c) Improved bistable switch design incorporating binding competition, along with positive feedback loops. Each TALE activator controls the expression of its own gene and the corresponding repressor gene, while the latter inhibits the expression of the opposing ranch with TALE activator and repressor. (d) A stochastic model of the switch with a positive feedback loop. Modelling determined that the improved design should be able to adopt one of the two stable states and toggle between them on the input signal pulse. The details of the model are available inSupplementary Note 2. PI and ER stand for pristinamycin and erythromycin, respectively. The magenta and green lines indicate the calculated TagBFP and mCitrine reporter gene expression levels, respectively. Full size image Figure 3: Introduction of nonlinearity into a genetic circuit based on monomeric DNA-binding elements employing competition and positive feedback loops. ( a ) A TALE repressor and a TALE activator based on the same DNA-binding domain competing for binding to the same DNA target site. ( b ) The competition of the TALE-based activator and repressor for the same binding site was experimentally tested using the luciferase reporter. Various ratios of plasmids constitutively expressing a TALE activator and a TALE repressor based on the same DNA-binding domain were co-transfected into HEK293T cells, along with 75 ng of the corresponding reporter plasmid, which resulted in different levels of the expression of the reporter. The values represent the mean and s.d. of three replicates and are representative of at least three independent experiments. Fit of the model based on parameters extracted from the experimental data of all experiments overlays the experimental data. ( c ) Improved bistable switch design incorporating binding competition, along with positive feedback loops. Each TALE activator controls the expression of its own gene and the corresponding repressor gene, while the latter inhibits the expression of the opposing ranch with TALE activator and repressor. ( d ) A stochastic model of the switch with a positive feedback loop. Modelling determined that the improved design should be able to adopt one of the two stable states and toggle between them on the input signal pulse. The details of the model are available in Supplementary Note 2 . PI and ER stand for pristinamycin and erythromycin, respectively. The magenta and green lines indicate the calculated TagBFP and mCitrine reporter gene expression levels, respectively. Full size image Maintenance of the stability in a TALE-based genetic switch For the experimental implementation of the bistable switch, we combined the positive feedback loops and competition effects into the same circuit ( Fig. 3c ). This circuit topology requires only one pair of designed DNA-binding (TALE) domains to construct two repressor–activator pairs, requiring only one DNA operator sequence for each of the two branches of the switch device. Deterministic ( Supplementary Fig. 3 and Supplementary Note 1 ) and stochastic ( Fig. 3d ) system analysis showed that the switch design that incorporated positive feedback loops with an activator and binding competition performed best. The state of the switch was regulated externally by the same pair of chemical inducers (pristinamycin and erythromycin) used for the mutual repressor switch, with the addition of two TALE activators under the control of chemically inducible transcription factors ( Fig. 4a and Supplementary Fig. 4 ). Both inducible systems, when coupled with TALE activators ( Supplementary Fig. 2c,e ), exhibited low leakage and high differences in the reporter activity between the stimulated and unstimulated states ( Supplementary Fig. 2d,f ). Experiments on the activation of individual branches of the switch provided parameter values to model the optimal ratio of the activator/repressor operons ( Fig. 5 and Supplementary Note 2 ) and test the experimental implementation of the competitive feedback switch. In principle, an activator and repressor targeted against different binding sites could also be joined in a single t2A sequence-linked reading frame. However, simulations demonstrated that the separate operons provide an additional tool for tuning the performance of the switch that the optimal ratio of activator versus repressor is different from 1:1. 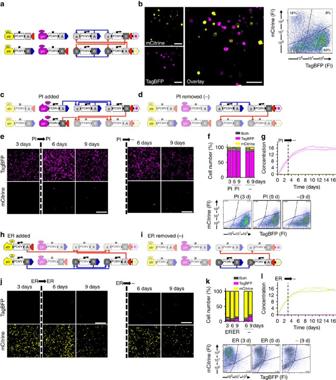Figure 4: The improved design of the TALE-based bistable genetic switch displays bistability. (a) Introduction of binding competition, along with positive feedback loops, into the TALE-based mutual repressor switch. The TALE activators contain the same DNA-binding domains as the TALE repressors of the opposite state. External control was provided in the same fashion as for the mutual repressor switch (Fig. 1b), with the addition of two inducer-dependent TALE activator operons. (b) Confocal microscopy and flow cytometry analyses of the TALE-based competitive feedback switch in the absence of external regulation demonstrate bimodal fluorescence distribution. Cells expressing either a TagBFP or mCitrine reporter are marked magenta or yellow, respectively. Scale bar, 50 μm. Schematic presentation of the pristinamycin (PI) (c) and erythromycin-induced (ER) (h) state, and the subsequent stable state on PI (d) and ER removal (i). Confocal microscopy (e,j) and flow cytometry (f,k) analyses of the PI-induced and stable (−) states (e,f) and of the ER-induced and stable (−) states (j,k). Scale bar, 250 μm. The fraction of cells expressing specific reporters obtained from flow cytometry is presented in the histograms. (g,l) Stochastic modelling determined that the improved design is able to retain a stable state, even after the removal of an inducer: (g) removal of pristinamycin (PI to ‘−’) and (l) erythromycin (ER to ‘−’) as described inSupplementary Note 2. Magenta and green lines indicate the calculated TagBFP and mCitrine reporter gene expression levels, respectively. Results are representative of at least three independent experiments. Figure 4: The improved design of the TALE-based bistable genetic switch displays bistability. ( a ) Introduction of binding competition, along with positive feedback loops, into the TALE-based mutual repressor switch. The TALE activators contain the same DNA-binding domains as the TALE repressors of the opposite state. External control was provided in the same fashion as for the mutual repressor switch ( Fig. 1b ), with the addition of two inducer-dependent TALE activator operons. ( b ) Confocal microscopy and flow cytometry analyses of the TALE-based competitive feedback switch in the absence of external regulation demonstrate bimodal fluorescence distribution. Cells expressing either a TagBFP or mCitrine reporter are marked magenta or yellow, respectively. Scale bar, 50 μm. Schematic presentation of the pristinamycin (PI) ( c ) and erythromycin-induced (ER) ( h ) state, and the subsequent stable state on PI ( d ) and ER removal ( i ). Confocal microscopy ( e , j ) and flow cytometry ( f , k ) analyses of the PI-induced and stable (−) states ( e , f ) and of the ER-induced and stable (−) states ( j , k ). Scale bar, 250 μm. The fraction of cells expressing specific reporters obtained from flow cytometry is presented in the histograms. ( g , l ) Stochastic modelling determined that the improved design is able to retain a stable state, even after the removal of an inducer: ( g ) removal of pristinamycin (PI to ‘−’) and ( l ) erythromycin (ER to ‘−’) as described in Supplementary Note 2 . Magenta and green lines indicate the calculated TagBFP and mCitrine reporter gene expression levels, respectively. Results are representative of at least three independent experiments. 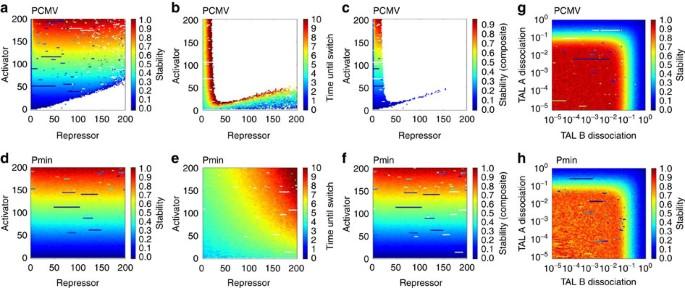Figure 5: The minimal promoter competitive feedback switch is more robust to variations in the repressor:activator ratio than the switch based on the constitutive (cytomegalovirus (CMV)) promoter. Parameter scans of stochastic topology models regarding the concentration of activator and repressor. The evaluation criteria were calculated after 17 simulation days. Stability is defined asR2—R1, whereR2is the concentration of an induced state reporter andR1is the concentration of the repressed state reporter. This criterion is normalized for its maximal value across the scanned region. The first inducer was introduced att0=0 and removed aftert1=3 days. The time until the switch is defined ast2−t1(in number of days), wheret1represents the time of the second inducer introduction andt2the time until theR2concentration becomes larger thanR1. The first inducer was introduced att0=0 and the second inducer att1=3 days. White areas represent parameter values for which the simulations predict instability (negative stability value) and/or the inability to switch between the states (R2never becomes greater thanR1). Amounts of activators and repressors were varied as dosage of the constructs PMIN/CMVA0, PMIN/CMVB0, PCMVPIP0, PCMVE0and PMIN/CMVA1, PMIN/CMVB1, PCMVPIP1, PCMVE1. Details on the constructs are available inSupplementary Tables 8 and 9. (a,b) Evaluation of the stability and state switching ranges for the CMV promoter competitive feedback switch (Fig. 2c). Simulations indicate that toggling between states is possible only within a narrow range of repressor:activator ratios for topology based on PCMV. (c) Composite image ofaandb, displaying the range of robust stability and switching. (d,e) Evaluation of stability and state switching ranges for the minimal promoter competitive feedback switch (Fig. 5a). The range of positive stability and state switching is significantly wider than for the CMV promoter competitive feedback switch (a,b), displaying higher robustness to variations in the activator:repressor ratios. (f) Composite image ofdande, displaying range robust stability and switching. Details on the model are available inSupplementary Note 2. (g,h) Scan of the effect of the affinities of the TALE-binding domains displaying the similar effect on stability of both types of switches. Full size image Figure 5: The minimal promoter competitive feedback switch is more robust to variations in the repressor:activator ratio than the switch based on the constitutive (cytomegalovirus (CMV)) promoter. Parameter scans of stochastic topology models regarding the concentration of activator and repressor. The evaluation criteria were calculated after 17 simulation days. Stability is defined as R 2 — R 1 , where R 2 is the concentration of an induced state reporter and R 1 is the concentration of the repressed state reporter. This criterion is normalized for its maximal value across the scanned region. The first inducer was introduced at t 0 =0 and removed after t 1 =3 days. The time until the switch is defined as t 2 − t 1 (in number of days), where t 1 represents the time of the second inducer introduction and t 2 the time until the R 2 concentration becomes larger than R 1 . The first inducer was introduced at t 0 =0 and the second inducer at t 1 =3 days. White areas represent parameter values for which the simulations predict instability (negative stability value) and/or the inability to switch between the states ( R 2 never becomes greater than R 1 ). Amounts of activators and repressors were varied as dosage of the constructs PMIN/CMV A0 , PMIN/CMV B0 , PCMV PIP0 , PCMV E0 and PMIN/CMV A1 , PMIN/CMV B1 , PCMV PIP1 , PCMV E1 . Details on the constructs are available in Supplementary Tables 8 and 9 . ( a , b ) Evaluation of the stability and state switching ranges for the CMV promoter competitive feedback switch ( Fig. 2c ). Simulations indicate that toggling between states is possible only within a narrow range of repressor:activator ratios for topology based on PCMV. ( c ) Composite image of a and b , displaying the range of robust stability and switching. ( d , e ) Evaluation of stability and state switching ranges for the minimal promoter competitive feedback switch ( Fig. 5a ). The range of positive stability and state switching is significantly wider than for the CMV promoter competitive feedback switch ( a , b ), displaying higher robustness to variations in the activator:repressor ratios. ( f ) Composite image of d and e , displaying range robust stability and switching. Details on the model are available in Supplementary Note 2 . ( g , h ) Scan of the effect of the affinities of the TALE-binding domains displaying the similar effect on stability of both types of switches. Full size image Cells harbouring the improved bistable switch device assumed a bimodal distribution in the absence of external induction, characterized by the expression of a single fluorescent reporter in the majority (60% TagBFP, 16% mCitrine and only 9% co-expressed both reporters) of the transfected individual cells ( Fig. 4b ). It has been previously observed that TALE domains can exhibit variations in terms of binding affinity [31] . The slightly stronger repression of TALB:KRAB compared with TALA:KRAB, as observed in the titration experiment ( Fig. 3b ), caused a strong bias (1:4) in the state selection in the absence of an inducer. Nevertheless, the overwhelming population of cells expressing a single reporter rather than both reporters simultaneously implied that such a system is bistable. Transient induction via either of the two chemical inducers shifted the system towards the expected state, with a very low level of expression of the opposing state ( Fig. 4c–f,h–k ). Despite the imbalance in the repression strength of the two TALE repressors, cells retained either of the two selected states equally well for more than 6 days after the chemical inducer was removed ( Fig. 4e,f,j,k ). This indicates that the improved switch design functions as predicted by the model ( Fig. 4g,l ). Modelling indicated that the system is insensitive to the several orders of magnitude of difference in DNA-binding strength between the pair of TALE domains due to the positive feedback loop ( Fig. 5 and Supplementary Note 2 ). Functional switching between stable states Although the improved switch topology retained the epigenetic state after the chemical inducer was removed, a functional bistable switch should also support controlled reversible toggling between the two stable states. We tested this property via the initial induction of one state, followed by the replacement with the second chemical inducer. Experimental results showed the expected trends in expression of the two reporters 6 days after the inducer replacement, but the emergence of the second state was too slow for the reliable confirmation ( Supplementary Fig. 5 ). To increase the difference between the levels of transcription for the repressed and activated states, the constitutive promoter of the core switch was replaced with a minimal promoter, which exhibits essentially no reporter gene expression in the absence of an activator or in the presence of a repressor. However, the minimal promoter setup could not be used for the basic toggle switch, as it requires repression. Modelling indicated that a system based on minimal promoters is more robust, that is, it is even less sensitive to the incomplete repression than the competitive feedback switch based on the constitutive promoter ( Fig. 5 and Supplementary Note 2 ) and is able to transition between the states more quickly ( Fig. 6 and Supplementary Fig. 6 ). 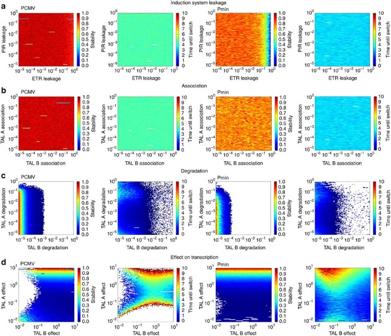Figure 6: Sensitivity of the improved bistable switch to different TALE-regulator-dependent parameters. Parameter scans of stochastic simulation of topology models based on Pmin or PCMV promoters as a function of the TALE regulator-dependent parameters. The simulation setting with evaluation criteria for stability and switching times is defined as inFig. 4. White areas represent parameter values for which the simulations predict instability (negative stability value) and/or the inability to switch between the states. Parameter labels refer toSupplementary Table 7. (a) Parameter scans of the leakage of the PIP/ETR induction systems (lCMV ). The parameter does not significantly change any evaluation criterion in either switch model. (b) Parameter scans of the leakage of the TALE association constants (kT). The parameter does not significantly change any evaluation criterion in either switch model. (c) Parameter scans of the TALE-A/TALE-B degradation rates (dT). The simulations predict a slightly higher stability and switching range of the switch based on PCMV. (d) Parameter scans of TALE-A/TALE-B effect on transcription. To account for variation in the TALE-A/TALE-B effect, the parameters were multiplied by factors, ranging from 10−2to 101, as shown on the parameter axes. The variation significantly affects the stability and the switching ability of the PCMV-based switch, while the PMIN variant displays higher robustness in this respect. Details on the models are available inSupplementary Note 2. Figure 6: Sensitivity of the improved bistable switch to different TALE-regulator-dependent parameters. Parameter scans of stochastic simulation of topology models based on Pmin or PCMV promoters as a function of the TALE regulator-dependent parameters. The simulation setting with evaluation criteria for stability and switching times is defined as in Fig. 4 . White areas represent parameter values for which the simulations predict instability (negative stability value) and/or the inability to switch between the states. 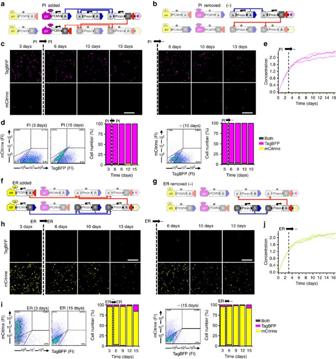Figure 7: The competitive feedback switch with minimal promoters exhibits state stability in the absence of an inducer. The presence of pristinamycin (PI) or erythromycin (ER) triggers expression of the selected state, as depicted in the schematic representation (a,f), and confirmed with confocal microscopy (c,h) and flow cytometry (d,i). Removal of the inducer molecule 3 days after transfection resulted in stable states as depicted in the schematic representation (b,g), and confirmed even after 13 days with confocal microscopy (c,h) and flow cytometry (d,i). The microscopy and flow cytometry results are representative of at least three independent experiments. Scale bar, 50 μm. The number of cells expressing specific reporters (as obtained from flow cytometry) is presented in the histograms. A stochastic model of the pristinamycin-induced state (e) or the erythromycin-induced state (j) results in state stability, matching the experimental results. Details on the model are available inSupplementary Note 2. Parameter labels refer to Supplementary Table 7 . ( a ) Parameter scans of the leakage of the PIP/ETR induction systems (lCMV ). The parameter does not significantly change any evaluation criterion in either switch model. ( b ) Parameter scans of the leakage of the TALE association constants (kT). The parameter does not significantly change any evaluation criterion in either switch model. ( c ) Parameter scans of the TALE-A/TALE-B degradation rates (dT). The simulations predict a slightly higher stability and switching range of the switch based on PCMV. ( d ) Parameter scans of TALE-A/TALE-B effect on transcription. To account for variation in the TALE-A/TALE-B effect, the parameters were multiplied by factors, ranging from 10 −2 to 10 1 , as shown on the parameter axes. The variation significantly affects the stability and the switching ability of the PCMV-based switch, while the PMIN variant displays higher robustness in this respect. Details on the models are available in Supplementary Note 2 . Full size image The experimental results of the switch based on the minimal promoter clearly demonstrated state stability even 12 days after the inducer was removed ( Fig. 7 ). Cells harbouring minimal promoter-based competitive feedback switch plasmids ( Fig. 8a ) assumed a bimodal distribution in the absence of external induction, characterized by the expression of a single fluorescent reporter in the majority (80% TagBFP, 19% mCitrine and only 1% co-expressed both reporters) of the individual cells expressing TagBFP or mCitrine ( Fig. 8b ). State transition was monitored from both initial conditions via the confocal microscopy and flow cytometry ( Fig. 7 ). However, some of the initial fluorescent reporter proteins remained after the transition, presumably due to the slow degradation of fluorescent proteins, making them a less suitable choice as reporters for dynamic experiments ( Supplementary Fig. 7 ). To overcome this drawback, we used a firefly luciferase reporter, which has a higher turnover rate instead. This final setup of the competitive feedback loop switch demonstrated successful multiple toggling of a TALE-based switch between the on and off states in both directions over the course of 17 days ( Fig. 8d–g ). Figure 7: The competitive feedback switch with minimal promoters exhibits state stability in the absence of an inducer. The presence of pristinamycin (PI) or erythromycin (ER) triggers expression of the selected state, as depicted in the schematic representation ( a , f ), and confirmed with confocal microscopy ( c , h ) and flow cytometry ( d , i ). Removal of the inducer molecule 3 days after transfection resulted in stable states as depicted in the schematic representation ( b , g ), and confirmed even after 13 days with confocal microscopy ( c , h ) and flow cytometry ( d , i ). The microscopy and flow cytometry results are representative of at least three independent experiments. Scale bar, 50 μm. The number of cells expressing specific reporters (as obtained from flow cytometry) is presented in the histograms. A stochastic model of the pristinamycin-induced state ( e ) or the erythromycin-induced state ( j ) results in state stability, matching the experimental results. Details on the model are available in Supplementary Note 2 . 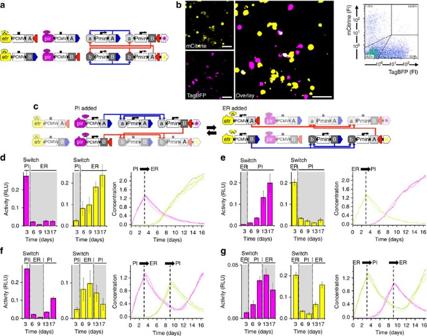Figure 8: Regulated transitions between the two stable states of the switch. (a) Introduction of minimal promoters into the TALE-based competitive feedback switch. The mutual TALE repressors and the corresponding TALE activators of the feedback loop are placed under the control of a minimal promoter. (b) Confocal microscopy analysis of the TALE-based competitive feedback switch in the absence of external regulation indicates bimodal distribution of fluorescent proteins. Cells expressing either a TagBFP or mCitrine reporter are marked in magenta or yellow, respectively. Cells expressing both reports at the same time (3%) are marked white on the overlay image. Scale bar, 50 μm. (c) Schematic representation of toggling between the pristinamycin (PI)- and erythromycin (ER)-induced states. (d–g) Switching between stable states was experimentally tested using luminometry (mean with s.d.,n=4). The purple bar graphs represent firefly luciferase activity in a switch in which the luciferase gene was used to replace the TagBFP reporter, while the yellow bar graphs correspond to the version with the luciferase gene replacing the mCitrine reporter. Switching between the states was tested in both directions, (d) pristinamycin–erythromycin (PI→ER) and (e) erythromycin–pristinamycin (ER→PI), as well as for multiple switch events: (f) pristinamycin–erythromycin–pristinamycin and (g) erythromycin–pristinamycin–erythromycin. Experimental results are in agreement with the stochastic models (shown on the right side of the panels) and demonstrate transitions between the on and off states depending on the presence of the selected chemical inducer as described inSupplementary Note 2. Results are representative of at least three independent experiments. Full size image Figure 8: Regulated transitions between the two stable states of the switch. ( a ) Introduction of minimal promoters into the TALE-based competitive feedback switch. The mutual TALE repressors and the corresponding TALE activators of the feedback loop are placed under the control of a minimal promoter. ( b ) Confocal microscopy analysis of the TALE-based competitive feedback switch in the absence of external regulation indicates bimodal distribution of fluorescent proteins. Cells expressing either a TagBFP or mCitrine reporter are marked in magenta or yellow, respectively. Cells expressing both reports at the same time (3%) are marked white on the overlay image. Scale bar, 50 μm. ( c ) Schematic representation of toggling between the pristinamycin (PI)- and erythromycin (ER)-induced states. ( d – g ) Switching between stable states was experimentally tested using luminometry (mean with s.d., n =4). The purple bar graphs represent firefly luciferase activity in a switch in which the luciferase gene was used to replace the TagBFP reporter, while the yellow bar graphs correspond to the version with the luciferase gene replacing the mCitrine reporter. Switching between the states was tested in both directions, ( d ) pristinamycin–erythromycin (PI→ER) and ( e ) erythromycin–pristinamycin (ER→PI), as well as for multiple switch events: ( f ) pristinamycin–erythromycin–pristinamycin and ( g ) erythromycin–pristinamycin–erythromycin. Experimental results are in agreement with the stochastic models (shown on the right side of the panels) and demonstrate transitions between the on and off states depending on the presence of the selected chemical inducer as described in Supplementary Note 2 . Results are representative of at least three independent experiments. Full size image Designable modular DNA-binding domains provide a powerful enrichment of the toolbox for the rational regulation of biological processes [21] , [32] , [33] . The already demonstrated ability to generate tens of thousands of designed DNA-binding domains targeting different DNA sequences [34] , [35] represents the great potential for the designed regulatory circuits of increased complexity and orthogonality. In this report we show that in addition to the static logic circuits, designable DNA-binding domains can be used to construct dynamic logic devices. Here we present a general strategy for implementing the designed DNA-binding domains to construct bistable switches, which has strong scaling potential due to the modularity and orthogonality. The main feature of our design is the introduction of a nonlinear response, which is required to construct complex dynamic regulatory circuits, through the introduction of positive feedback loops and competition between the activator and the repressor for binding to the same DNA operator site. Competition and feedback loops in transcriptional regulatory circuits have been already analysed previously [36] , [37] ; however, those designs incorporated cooperative transcriptional regulators or regulator features that would be very difficult to implement experimentally. The design of a bistable switch based on linear response elements has been experimentally demonstrated in a few special cases, such as using a T7 RNA polymerase that activates its own expression. In that case, the retardation of cell growth due to the circuit activation caused nonlinear dilution of the T7 RNA polymerase in individual bacteria, which, combined with the feedback, resulted in bistability [38] . A bistable switch with non-cooperative elements has also been demonstrated based on sequestration and positive feedback using sigma and anti-sigma factors [39] . In contrast to those designs, which are based on few selected biological phenomena or molecules, our platform is based on an extremely large pool of orthogonal DNA-binding elements that can be applied to the design of multiple orthogonal switches that could operate within the same cell or more complex switches. As a demonstration we designed a tristable switch based on three different inputs, which is an extension of a bistable switch and also involves the positive feedback loop and competition ( Fig. 9 ). In addition, the tools developed in this report allow design of a tristable switch, regulated by different combinations of only two input signals ( Fig. 10 ). This switch device requires four TALE-binding domains to build a topology that can distinguish between the first, second or both input channel pulses simultaneously and allows reversible switching between any combinations, extending the ability to control cell states. Simulation of those switches based on the parameters from an experimentally verified bistable TALE-based switch indicates that the design of those more complex switches is functional. The designable orthogonal DNA-binding modules allow the construction of parallel orthogonal bistable switches within a single cell, requiring only one pair of orthogonal designed DNA-binding domains per bit of cellular memory. With the ability to massively generate different TALE domains or sgRNA/Cas combinations for the CRISPR system, the design presented here therefore expands the potential regulatory and memory capacity of biological systems. Different input signals from the environment or internal cellular processes (for example, cell type-characteristic transcription factors [40] ) that could be converted into the transcriptional signal could be used to regulate the designed circuits for different applications, for example, sensing or therapeutic. 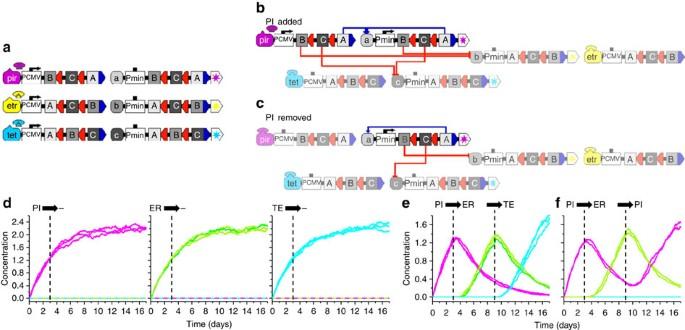Figure 9: Design of a tristable genetic transcription circuit regulated by three different input signals. (a) Schematic representation of the circuit components comprising three pairs of chemical inducer sensitive regulators, combinations of two repressors that repress transcription of two other constructs and an activator that activates its own transcription; (b) state of the switch in the presence of one chemical inducer (PI). Other two states are regulated in the same manner. (c) State of the switch when the particular inducer has been removed. (d) Stochastic simulation of the switch in the presence of each inducer for 3 days and its removal afterward demonstrates the stability of the circuit. (e) Simulation of switching from the pristinamycin- to the erythromycin-induced state, followed by switching to the tetracyclin-induced state (PI→ER→TET). (f) Simulation of switching from the pristinamycin- to the erythromycin-induced state, followed by switching back to the pristinamycin-induced state (PI→ ER→PI). The design enables toggling between all three states, regardless of their order and the initial state. Details on the model are available inSupplementary Note 2. Figure 9: Design of a tristable genetic transcription circuit regulated by three different input signals. ( a ) Schematic representation of the circuit components comprising three pairs of chemical inducer sensitive regulators, combinations of two repressors that repress transcription of two other constructs and an activator that activates its own transcription; ( b ) state of the switch in the presence of one chemical inducer (PI). Other two states are regulated in the same manner. ( c ) State of the switch when the particular inducer has been removed. ( d ) Stochastic simulation of the switch in the presence of each inducer for 3 days and its removal afterward demonstrates the stability of the circuit. ( e ) Simulation of switching from the pristinamycin- to the erythromycin-induced state, followed by switching to the tetracyclin-induced state (PI→ER→TET). ( f ) Simulation of switching from the pristinamycin- to the erythromycin-induced state, followed by switching back to the pristinamycin-induced state (PI→ ER→PI). The design enables toggling between all three states, regardless of their order and the initial state. Details on the model are available in Supplementary Note 2 . 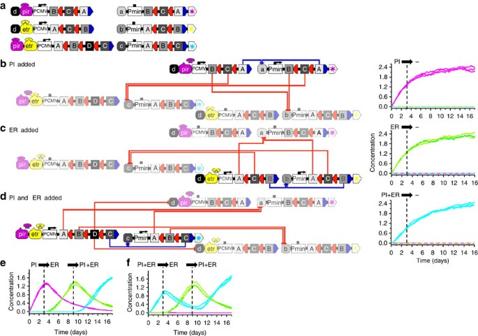Figure 10: Design of a tristable genetic transcription circuit regulated by different combinations of two input signals. (a) Schematic representation of the circuit components, comprising four TALE-based activators, repressors and their binding sites. State 3 is induced in the presence of two inducers simultaneously. As the presence of both inducers can potentially induce each of the three states, an additional TALE repressor is included (TALE-D) to repress induction system constructs for pristinamycin- and erythromycin-induced states; (b–d) states of the switch in the presence of PI, ER and both PI and ER, respectively. Simulations (right panels) represent states in the presence of the appropriate inducers for three days and their removal afterwards; (e) switching from the pristinamycin- to the erythromycin-induced state, followed by the addition of pristinamycin and erythromycin (PI→ER→PI+ER); (f) switching from the two inducer-induced state to the erythromycin-induced state and back to the two inducer-induced state (PI+ER → ER→PI+ER). The design enables toggling between all three possible states, regardless of their order and the initial state. The transition from the two inducer-induced state is possible regardless of the additional TALE-D repressor presence. Details on the model are available inSupplementary Note 2. Full size image Figure 10: Design of a tristable genetic transcription circuit regulated by different combinations of two input signals. ( a ) Schematic representation of the circuit components, comprising four TALE-based activators, repressors and their binding sites. State 3 is induced in the presence of two inducers simultaneously. As the presence of both inducers can potentially induce each of the three states, an additional TALE repressor is included (TALE-D) to repress induction system constructs for pristinamycin- and erythromycin-induced states; ( b – d ) states of the switch in the presence of PI, ER and both PI and ER, respectively. Simulations (right panels) represent states in the presence of the appropriate inducers for three days and their removal afterwards; ( e ) switching from the pristinamycin- to the erythromycin-induced state, followed by the addition of pristinamycin and erythromycin (PI→ER→PI+ER); ( f ) switching from the two inducer-induced state to the erythromycin-induced state and back to the two inducer-induced state (PI+ER → ER→PI+ER). The design enables toggling between all three possible states, regardless of their order and the initial state. The transition from the two inducer-induced state is possible regardless of the additional TALE-D repressor presence. Details on the model are available in Supplementary Note 2 . Full size image In conclusion, orthogonally designed DNA-binding domains can be used for the dynamic cell regulation through constructing multistable genetic switches. The availability of a very large number of designable orthogonal DNA-binding domains represents the foundation for the construction of parallel orthogonal switches, each requiring only two DNA-binding domains to assume the selected epigenetic memory states. The introduction of nonlinearity into the system based on linear response–regulatory elements based on the principles used here could be applied to other biological information mediators that exhibit non-cooperative binding, particularly for other modular DNA-binding domains, such as zinc fingers, CRISPR/Cas or helix-coil-helix domains. Finally, although this type of regulation has been demonstrated in mammalian cells, it is transferable to other cell chassis through the use of appropriate activation/repression domain modules. Plasmid construction All plasmids used were constructed with classic molecular cloning methods or the Gibson assembly method [41] and are listed in Supplementary Table 1 . The nucleotide and amino acid sequences are provided in Supplementary Table 2 . The TALE DNA-binding domains (TALA, aa 2–804 and TALB, aa 2–804) were PCR amplified from TALEN1257 (plasmid 32280, Addgene) and TALEN1297 (plasmid 32279, Addgene) [42] , respectively. The KRAB domain was obtained from pLVPT-rtTR-KRAB-2SM2 (plasmid 11652, Addgene) [43] and the VP16 domain was obtained from the vector pSGVP, which was provided by Professor Dr Mark Ptashne (Memorial Sloan Kettering Cancer Center, New York, NY, USA) [44] . TALA and TALB operators [21] were designed as multiple repeats of their target sequences, separated by hypervariable linkers, and synthesized by Life Technologies. Erythromycin- and pristinamycin-dependent DNA-binding proteins E and PIP (plasmids pWW35 and pMF207), as well as the corresponding DNA-binding sites etr and pir (plasmids pWW56 and pMF208), were provided by Professor Dr Martin Fussenegger (Department of Biosystems Science and Engineering, ETH Zürich, Switzerland) [25] , [26] . The reporter genes were PCR amplified from commercial plasmids: firefly luciferase from pGL4.16 (Promega), TagBFP from pTagBFP-N (Evrogen) and mCitrine [45] obtained as a gift from Dr Oliver Griesbeck (the Max Planck Institute of Neurobiology, Munchen, Germany). Renilla luciferase (phRL-TK, Promega), mCherry (pmCherry-C1, Clontech) and iRFP670 (ref. 46 ) (synthesized by Life Technologies) were used as the transfection controls. The SV40 large T-antigen nuclear localization sequence, the hexa-histidine tag and the t2A sequence [47] were introduced into the constructs with PCR. Cell culture The human embryonic kidney (HEK) 293 T cell line (American Type Culture Collection, Manassas, VA, USA) was cultured in DMEM medium (Invitrogen) supplemented with 10% fetal bovine serum) (BioWhittaker, Walkersville, MD, USA) at 37 °C in a 5% CO 2 environment. Inducer molecules Erythromycin (Sigma-Aldrich) and pristinamycin (Sanofi-Aventis) were prepared as stock solutions of 50 mg ml −1 (erythromycin in ethanol, pristinamycin in dimethyl sulphoxide) and used at a final concentration of 2 μg ml −1 . Luciferase reporter assay HEK293T cells (2 × 10 4 cells per well) were seeded in CoStar White 96-well plates (Corning). At 50–70% confluence, they were transfected with a mixture of DNA and JetPEI according to the manufacturer’s instructions (Polyplus-transfection). Every 3 days, the cells were supplemented with fresh medium and (where appropriate) inducer molecules. At various time points, the cells were harvested and lysed with 30 μl of 1 × passive lysis buffer (Promega). Firefly luciferase and Renilla luciferase expression were measured using a dual luciferase assay (Promega) and an Orion II microplate reader (Berthold Technologies, Pforzheim, Germany). Relative luciferase activity was calculated by normalizing each sample’s firefly luciferase activity to the constitutive Renilla luciferase activity determined within the same sample. The graphs represent the mean and s.d. from the mean of at least three measurements within an experiment. The data are representative of at least three independent experiments. Flow cytometry HEK293T cells were seeded in 24-well plates (1 × 10 5 cells per well) or in 12-well plates (5 × 10 5 cells per well) (TPP, Trasadingen, Switzerland). At 50–70% confluence, they were transfected with a mixture of DNA and JetPEI according to the manufacturer’s instructions (Polyplus-transfection). Every 3 days, the cells were supplemented with fresh medium and (where appropriate) inducer molecules. At various time points, the cells were washed with ice-cold PBS and harvested with 500 μl of FACS buffer (3% fetal bovine serum in PBS). A flow cytometry analysis was performed with a CyFlow space flow cytometer (Partec, Münster, Germany). A 488-nm diode laser was used to detect mCitrine, a 405-nm diode laser was used to detect TagBFP and a 633-nm diode laser was used to detect the iRFP670 transfection control. In each sample, at least 30,000 cells were analysed and gated to iRFP670-positive cells. The collected data were processed using FlowJo software (TreeStar, Ashland, OR, USA). The data are representative of at least three independent experiments. Confocal microscopy HEK293T cells (5 × 10 4 cells per well) were seeded in eight-well tissue culture chambers (μ-Slide 8 well, Ibidi Integrated BioDiagnostics, Martinsried München, Germany). At 30–50% confluence, the cells were transfected with a mixture of DNA and JetPEI transfection reagent according to the manufacturer’s instructions (Polyplus-transfection). Every 3 days, the cells were supplemented with fresh medium and (where appropriate) inducer molecules. Microscopic images were acquired at various time points using the Leica TCS SP5 inverted laser-scanning microscope on a Leica DMI 6000 CS module equipped with a HCX PL Fluotar L 20 × , numerical aperture 0.4 (Leica Microsystems, Wetzlar, Germany). A 514-nm laser line of a 100-mW argon laser with 25% laser power was used for mCitrine excitation, and the emitted light was detected between 520 and 580 nm. A 50-mW 405-nm diode laser was used for TagBFP excitation and the emitted light was detected between 420 and 460 nm. A 1-mW 543-nm HeNe laser was used for mCherry excitation and the emitted light was detected between 560 and 630 nm. Leica LAS AF software was used for acquisition and ImageJ software was used for image processing. The data are representative of at least three independent experiments and five separate observations within each experiment. How to cite this article: Lebar, T. et al . A bistable genetic switch based on designable DNA-binding domains. Nat. Commun. 5:5007 doi: 10.1038/ncomms6007 (2014).